Coherent spin control of a nanocavity-enhanced qubit in diamond A central aim of quantum information processing is the efficient entanglement of multiple stationary quantum memories via photons. Among solid-state systems, the nitrogen-vacancy centre in diamond has emerged as an excellent optically addressable memory with second-scale electron spin coherence times. Recently, quantum entanglement and teleportation have been shown between two nitrogen-vacancy memories, but scaling to larger networks requires more efficient spin-photon interfaces such as optical resonators. Here we report such nitrogen-vacancy-nanocavity systems in the strong Purcell regime with optical quality factors approaching 10,000 and electron spin coherence times exceeding 200 μs using a silicon hard-mask fabrication process. This spin-photon interface is integrated with on-chip microwave striplines for coherent spin control, providing an efficient quantum memory for quantum networks. The coupling between photons and quantum states of an emitter is efficient in the strong Purcell regime, in which the emitter interacts primarily with one optical mode. This regime is reached when the overall Purcell enhancement exceeds one ( F >1) [1] . In the case of a nitrogen-vacancy (NV) centre, only a small fraction of the overall photoluminescence (PL) is emitted via the zero-phonon line (ZPL) transitions [2] . Therefore, one has to differentiate between the overall Purcell enhancement F and the spectrally resolved spontaneous emission (SE) rate enhancement F ZPL = F /DW, where DW is the Debye–Waller factor. When the NV ZPL is coupled to a cavity with quality factor Q and mode volume V mode , the enhancement is given by where is the maximum spectrally resolved SE rate enhancement [3] and quantifies the angular and spatial overlap between the dipole moment ( μ ) and the cavity mode electric field ( E ). A high can be realised in photonic crystal (PhC) nanocavities due to their small mode volumes [4] V mode ~( λ / n ) 3 and their large quality factors. One-dimensional (1D) and 2D PhC cavities in diamond [5] , [6] , [7] have reached Q factors of 6,000 and 3,000 and F ZPL up to 7 and 70, respectively. However, the only spin measurement demonstrated on a cavity-coupled NV showed a ~1 μs Rabi envelope decay from an NV hosted in a nanodiamond coupled to a gallium phosphide PhC cavity [8] . No spin coherence measurements have been reported on single-crystal diamond cavities, leaving unverified the potential of NV-cavity systems as quantum memories. Here we present a new fabrication scheme that enables exceptionally long-spin coherence times exceeding 200 μs, record-high nanocavity quality factors near the NV ZPL emission, as well as the demonstration of an NV in the strong Purcell regime with F ZPL of ~62. Our results experimentally validate the promise of long-spin coherence NV-cavity systems for scalable quantum repeaters and quantum networks. Simulation The cavities were designed using finite-difference time-domain simulations [9] to maximize by optimizing the ratio of Q / V mode ( Supplementary Fig. 1 and Supplementary Note 1 ). As shown in Fig. 1 , the nanocavity is based on a suspended 1D diamond PhC structure with lattice constant a , beam width w =2.4 a and thickness h =0.7 a . A linear increase of the lattice constant from 0.9 a to a in increments of 0.02 a per period away from the centre defines the cavity defect state. The fundamental cavity mode of the optimized structure yielded a simulated Q =6.02 × 10 5 and V mode =1.05( λ / n ) [3] . 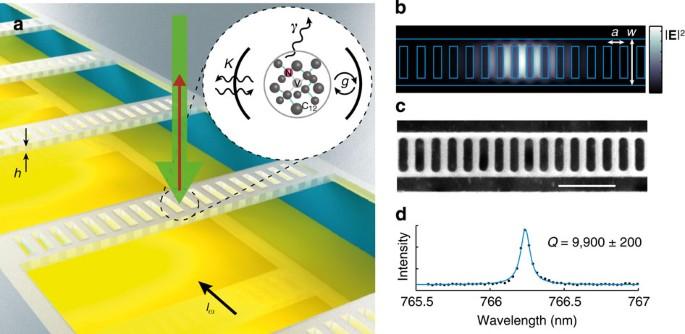Figure 1: On-chip NV-nanocavity system in diamond. (a) The diamond photonic crystal (PhC) cavities are integrated on a Si substrate with metallic striplines for coherent spin control and optically addressed using a confocal set up with 532 nm continuous-wave excitation and photoluminescence collected >630 nm. The inset shows the nitrogen-vacancy (NV)-nanocavity system withgthe NV-nanocavity Rabi frequency,γthe NV natural spontaneous emission (SE) decay rate andκthe cavity intensity decay rate. The NV consists of a substitutional nitrogen atom adjacent to a vacancy in the diamond lattice.Iωdenotes the current through the stripline, andhthe PhC thickness. (b) Simulated electric field intensity for the optimized fundamental cavity mode. The PhC has a widthWand a lattice constant varying from 0.9aat the centre toa=220 nm over five periods. (c) Scanning electron micrograph of a representative cavity structure. The scale bar represents 1 μm. (d) Measured cavity resonance (dots) with a quality factorQ~9,900±200 from a Lorentzian fit (blue line). Figure 1: On-chip NV-nanocavity system in diamond. ( a ) The diamond photonic crystal (PhC) cavities are integrated on a Si substrate with metallic striplines for coherent spin control and optically addressed using a confocal set up with 532 nm continuous-wave excitation and photoluminescence collected >630 nm. The inset shows the nitrogen-vacancy (NV)-nanocavity system with g the NV-nanocavity Rabi frequency, γ the NV natural spontaneous emission (SE) decay rate and κ the cavity intensity decay rate. The NV consists of a substitutional nitrogen atom adjacent to a vacancy in the diamond lattice. I ω denotes the current through the stripline, and h the PhC thickness. ( b ) Simulated electric field intensity for the optimized fundamental cavity mode. The PhC has a width W and a lattice constant varying from 0.9 a at the centre to a =220 nm over five periods. ( c ) Scanning electron micrograph of a representative cavity structure. The scale bar represents 1 μm. ( d ) Measured cavity resonance (dots) with a quality factor Q ~9,900±200 from a Lorentzian fit (blue line). Full size image Nanofabrication using silicon masks The cavities were patterned in high-purity single-crystal diamond using a new fabrication process that employs silicon (Si) membranes as etch masks. The diamond was fabricated by microwave (MW) plasma-assisted chemical vapour deposition (CVD), polished to 5 μm thickness and finally thinned to ~200 nm using a combination of chlorine- and oxygen-reactive ion etching (Methods). NVs were created by implantation of 15 N and subsequent annealing ( Fig. 2a ). The Si masks were produced by electron beam lithography and cryogenic plasma etching (sulfur hexafluoride and oxygen) from Si-on-insulator wafers with ~220-nm thick device layers [10] . This resulted in high-quality masks ~100 × 100 μm 2 in area. These were subsequently placed onto the diamond membranes using a transfer process described in the Methods ( Fig. 2b ). This Si mask transfer process enables nano-patterning without the need of resist coating onto the substrate and is compatible with sample sizes down to several tens of square micrometers. We used oxygen plasma [11] to etch the Si mask pattern into the pre-thinned ~200-nm diamond membranes ( Fig. 2c ). After mask removal, the patterned diamond membranes were transferred onto a Si chip with integrated MW striplines ( Fig. 2d ). Because the Si mask can be fabricated with excellent quality, thanks to the availability of mature fabrication technology for this material, this process yields diamond PhCs with low surface roughness and uniform, vertical sidewalls. We observed a high yield (94%) of cavities with resonances close to NV ZPL in a single fabrication run, with a maximum Q of 9,900±200 ( Fig. 2e ). Cavity resonances spectrally <637 nm are suitable for NV ZPL coupling via gas deposition tuning, while longer wavelength resonances can be blue detuned by thermal oxidation and oxygen plasma etching [5] , [7] . 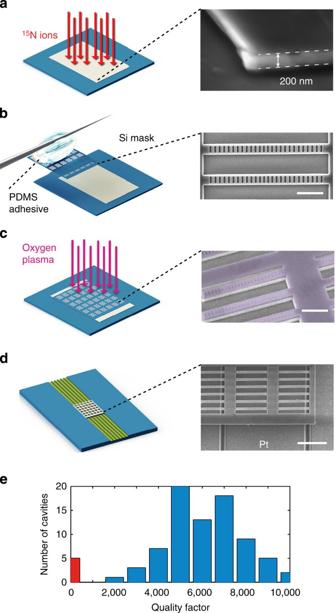Figure 2: Fabrication procedure and cavity characterization outcome. (a) NVs were created ~100 nm below the surface of the diamond membranes by implantation of15N atoms and subsequent annealing at 850 °C. The magnified scanning electron micrograph (SEM) shows a ~200 nm membrane. (b) Silicon (Si) masks were patterned on silicon-on-insulator, released and transferred onto diamond membranes. The SEM shows a patterned Si mask before transfer. The scale bar represents 1 μm. (c) Oxygen reactive ion etching was used to pattern diamond membranes. The false-colour SEM shows the Si mask (purple) on diamond after oxygen etching. The scale bar represents 1 μm. (d) Patterned diamond membrane on microwave striplines for optical and spin characterization. The SEM shows diamond PhC structures alongside metallic striplines in Si channels. The scale bar represents 5 μm. (e) Distribution of cavityQfactors from one fabrication run. Seventy-eight (blue bars) of 83 cavities showed resonances in the range of 600–770 nm, while 5 (red bar) showed no resonances in this wavelength range. Figure 2: Fabrication procedure and cavity characterization outcome. ( a ) NVs were created ~100 nm below the surface of the diamond membranes by implantation of 15 N atoms and subsequent annealing at 850 °C. The magnified scanning electron micrograph (SEM) shows a ~200 nm membrane. ( b ) Silicon (Si) masks were patterned on silicon-on-insulator, released and transferred onto diamond membranes. The SEM shows a patterned Si mask before transfer. The scale bar represents 1 μm. ( c ) Oxygen reactive ion etching was used to pattern diamond membranes. The false-colour SEM shows the Si mask (purple) on diamond after oxygen etching. The scale bar represents 1 μm. ( d ) Patterned diamond membrane on microwave striplines for optical and spin characterization. The SEM shows diamond PhC structures alongside metallic striplines in Si channels. The scale bar represents 5 μm. ( e ) Distribution of cavity Q factors from one fabrication run. Seventy-eight (blue bars) of 83 cavities showed resonances in the range of 600–770 nm, while 5 (red bar) showed no resonances in this wavelength range. Full size image Optical characterization We optically characterized samples at ambient and cryogenic (~18 K) temperatures using home-built confocal microscope set ups with 532 nm continuous-wave laser excitation. PL imaging ( Fig. 3a ) was used to identify NVs spatially within cavity centres, and spectral measurements determined the separation between the NV ZPL transitions and cavity resonances. Cavity system A (circled in Fig. 3a ) contains a single NV, as verified by antibunching in the second-order autocorrelation function. 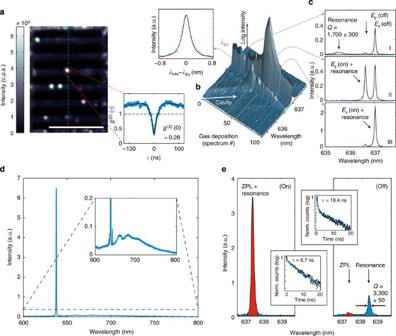Figure 3: Optical characterization of NV-nanocavity systems. (a) Photoluminescence confocal image of diamond PhC structures. The scale bar represents 5 μm. Single NVs are identified by circular white spots. System A: the dotted red circle shows a single NV close to the cavity centre (indicated by the blue dotted line). Inset: normalized second-order auto-correlation measurement withg(2)(0)=0.28. (b) Gas tuning of system A. The logarithmic plot shows the cavity resonance and two strain-split ZPL branches from a single NV (EyandEx, 2Δ=286 GHz, seeFig. 4a). As the gas condensation red shifts the cavity resonance, it sequentially enhances the two ZPL branches. The inset shows the intensity of theExZPL transition as a function of cavity detuning. This curve follows the expected Lorentzian dependence of the Purcell enhancement given by equation 1, and shows that the cavityQfactor remains constant throughout the tuning process. (c) Spectra of system A in the uncoupled (I) and coupled cases with(II) and(III). Note the difference in scaling betweenExandEycases. The black lines are Lorentzian fits to the data, yieldingQ=1,700±300 for the cavity. (d) System B at maximum Purcell enhancement. The inset shows a close-up of the spectrum. The ZPL transitions of four individual NVs (including the cavity-coupled ZPL) are visible, each with a different strain-induced spectral position. The accumulated phonon sidebands of these NVs are also apparent. (e) High resolution spectra of system B in cavity-coupled and uncoupled cases. The insets show the lifetime measurements corresponding toτon=6.7 ns andτoff=18.4 ns. Norm., normalized. Figure 3b,c plots the initial PL spectrum of system A, showing a cavity peak ( Q =1,700±300) blue detuned from the ZPL, as well as two ZPL branches E x and E y . These are split by 286 GHz due to local strain in the diamond lattice [12] . As shown in Fig. 3b , the cavity resonance was then gradually red shifted by gas deposition [13] to overlap with the NV ZPL transitions, resulting in strong PL enhancements (Methods). To determine F ZPL , a rate equation model is used to analyze the transition dynamics of the NV centre ( Supplementary Fig. 2 and Supplementary Note 2 ). In this simplified five-level model, we account for the SE rates of the phonon side-band (PSB) transitions and the different ZPL transition rates for the on- and off-resonance cases. The zero-phonon excited state to ground state transition rates of the NV are assumed to be enhanced by the factor F ZPL . One important input parameter of our model is the fraction of ZPL to total intensity, quantified by the DW factor [2] , which we estimate from an off-resonance spectrum to be DW=0.028. By substituting this factor into the rate equation model, we determine F ZPL of 8 (15) for transition E x ( E y ) in system A. To show that our simplified rate equation model gives a reliable prediction of F ZPL , we considered a second analysis method. By comparing the ZPL intensity for coupled and uncoupled cases ( Fig. 3c ), we can determine the ZPL SE coupling efficiency into the cavity mode parameterized by a factor , where is the intensity of the cavity-enhanced ZPL and I PSB is the intensity of the PSB. This method is valid in the weak excitation limit where the low population of the excited state does not influence the ratio of , where is the overall PL intensity when the NV ZPL is on resonance and is the overall PL intensity when the NV ZPL is off resonance (see Supplementary Note 2 ). From F ~ β /(1− β ), we can then deduce the increase in SE rate F ZPL = F /DW=10 (17) for the E x ( E y ) transition, yielding similar values compared with the rate equation analysis. Figure 3: Optical characterization of NV-nanocavity systems. ( a ) Photoluminescence confocal image of diamond PhC structures. The scale bar represents 5 μm. Single NVs are identified by circular white spots. System A: the dotted red circle shows a single NV close to the cavity centre (indicated by the blue dotted line). Inset: normalized second-order auto-correlation measurement with g (2) (0)=0.28. ( b ) Gas tuning of system A. The logarithmic plot shows the cavity resonance and two strain-split ZPL branches from a single NV ( E y and E x , 2Δ=286 GHz, see Fig. 4a ). As the gas condensation red shifts the cavity resonance, it sequentially enhances the two ZPL branches. The inset shows the intensity of the E x ZPL transition as a function of cavity detuning. This curve follows the expected Lorentzian dependence of the Purcell enhancement given by equation 1, and shows that the cavity Q factor remains constant throughout the tuning process. ( c ) Spectra of system A in the uncoupled (I) and coupled cases with (II) and (III). Note the difference in scaling between E x and E y cases. The black lines are Lorentzian fits to the data, yielding Q =1,700±300 for the cavity. ( d ) System B at maximum Purcell enhancement. The inset shows a close-up of the spectrum. The ZPL transitions of four individual NVs (including the cavity-coupled ZPL) are visible, each with a different strain-induced spectral position. The accumulated phonon sidebands of these NVs are also apparent. ( e ) High resolution spectra of system B in cavity-coupled and uncoupled cases. The insets show the lifetime measurements corresponding to τ on =6.7 ns and τ off =18.4 ns. Norm., normalized. Full size image These rate enhancements are still lower than theoretically expected, as determined by the Q and the transverse-electric (TE) polarization of the cavity mode. This is because the Purcell enhancement depends strongly on the spatial and angular overlap, and F ZPL is generally much lower than the maximum possible value, , especially in samples with low NV density (~1 NV per μm 2 in the case of system A). Moreover, for the {100} diamond crystal used here, the maximum Purcell enhancement is reduced to , since 35.3° is the smallest angle between the TE-cavity field and the NV dipole (that is, crystal) orientation. Using the rate equation model for system A, we calculate an overlap factor for transition E x ( E y ), indicating a factor of 1/ ξ ~10 (6) off from the theoretically expected maximum for our cavity design due to the non-ideal spatial and polarization overlap. The difference in ξ between E x and E y is attributed to different orientations of the two orthogonal NV dipoles with respect to the TE-cavity mode [14] . To reduce the deviation from the theoretical maximum and to investigate NV-nanocavity systems in the strong Purcell regime where >50% of the emission is coupled into a cavity mode, we studied another sample with the same cavity designs and a higher density of NVs (~10 μm −2 ). Figure 3d shows the PL spectrum of NV-nanocavity system B with Q B =3,300±50. Out of four ZPL transitions, one was strongly enhanced by the cavity mode; we attribute the remaining ZPL transitions to spatially decoupled NV centres within the ~2-μm diameter microscope collection spot through the cryostat window. We observed both a change in SE lifetime from the off-resonant case τ off ~18.4 ns to the on-resonant case τ on ~6.7 ns and a strong increase in emission from this NV ZPL when tuned onto resonance with the cavity ( Fig. 3d,e ). Due to the presence of multiple ZPL transitions and their accumulated PSBs, we cannot measure directly their individual DW factors, which are required to precisely determine the SE rate enhancement F ZPL as a function of DW. We therefore used two independent measurements to determine F ZPL and DW: (i) the rate equation model (as done for system A) and (ii) the radiative lifetime modification according to F ZPL =( τ bulk / τ on − τ bulk / τ off )/DW ( Fig. 3e ). Solving this system of equations gives F ZPL =62 and DW=0.019 for a measured τ bulk ~12.5 ns (the average lifetime of NVs in the un-patterned diamond membrane). The DW has been reported in a range from 0.01 to 0.19 at low temperature [2] , and has been shown to vary significantly with temperature shifts [15] ; because of this wide variability, we emphasize that it is important to obtain DW from separate measurements, as this strongly influences the estimated value of F ZPL . From a measured F ZPL of 62, we calculate a beta factor ( β ) of 0.54 which implies that the NV being enhanced is coupling >50% of its emission into one cavity mode. This value intuitively expresses that the overall NV emission was strongly redistributed towards the ZPL from 1.9 to 54%. Furthermore, by comparing our experimental enhancement to the theoretical expectation using the overlap factor , we find only threefold difference to the maximum value. Spin measurements The cavity-coupled NV centres exhibit excellent spin coherence times ( T 2 ) similar to the parent CVD crystal. 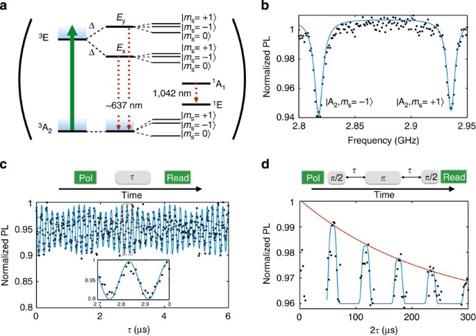Figure 4: Electronic structure and coherent spin control. (a) Energy level diagram of an NV centre in a nanocavity. The two excited state sublevels,ExandEy, are split by 2Δ~286 GHz due to strain in the lattice for NV system A (circled inFig. 3a). The effective SE rates of these excited states are modified by the nanocavity fromγto. For both the excited and ground state triplets, the |ms=0› and |ms=±1› states are split by the crystal field splitting, and the degeneracy of the |ms=±1› states is lifted by an applied magnetic field. (b) The optically detected magnetic resonance spectrum of the ground state triplet in NV system A with an applied field of ~2 mT. (c) By addressing only the transition between the |ms=0› and |ms=−1› states, we can coherently drive Rabi oscillations without observing any decay of the envelope function which indicates a>6 μs. The Rabi oscillations contain two frequency components, which we attribute to a hyperfine interaction with a nuclear spin. The inset above shows the Rabi sequence of polarization, pulsed microwave (MW) excitation and optical readout. (d) Using theπ/2 andπpulse durations from the Rabi measurement, we then applied a spin-echo sequence, determining theT2to be 230 μs. The inset above shows the Echo sequence of polarization, pulsedπ/2 andπMW pulses, and optical readout. Figure 4a shows the spin-preserving E x and E y optical transitions [14] of NV-nanocavity system A with associated magnetic sublevels m s =−1, 0,1. A small static magnetic field of ~2 mT was applied along the NV axis to lift the degeneracy of the m s =±1 spin states. The metastable spin singlet states ( E 1 , A 1 ) enable optically detected magnetic resonance (ODMR) measurements [14] , but we do not expect the transition rate between these levels to be modified by the cavity because the PhC bandgap, targeted near the ZPL at 637 nm, does not overlap with the 1,042 nm line. Figure 4b shows ODMR under continuous optical and MW excitation, indicating the m s =0→±1 spin transitions. Separate Rabi oscillation measurements ( Fig. 4c ) under pulsed excitation indicate a Rabi envelope decay time [16] of . (Please refer to Supplementary Fig. 3 and Supplementary Note 3 for T 1 measurements.) The phase coherence time F 2 is measured using a Hahn echo to cancel the dephasing by quasi-static magnetic fields [16] . From the single-exponential [17] decay envelope of the revivals in Fig. 4d , we estimate T 2 ~230 μs. Such T 2 values are typical for our parent high-purity electronic-grade diamond crystal, indicating that our novel Si mask nanofabrication process preserves long electron spin coherence times. This coherence time is more than 2 orders of magnitude longer than previously reported values for cavity-coupled NV centres [8] and semiconductor quantum dots [18] , [19] . Figure 4: Electronic structure and coherent spin control. ( a ) Energy level diagram of an NV centre in a nanocavity. The two excited state sublevels, E x and E y , are split by 2Δ~286 GHz due to strain in the lattice for NV system A (circled in Fig. 3a ). The effective SE rates of these excited states are modified by the nanocavity from γ to . For both the excited and ground state triplets, the | m s =0› and | m s =±1› states are split by the crystal field splitting, and the degeneracy of the | m s =±1› states is lifted by an applied magnetic field. ( b ) The optically detected magnetic resonance spectrum of the ground state triplet in NV system A with an applied field of ~2 mT. ( c ) By addressing only the transition between the | m s =0› and | m s =−1› states, we can coherently drive Rabi oscillations without observing any decay of the envelope function which indicates a >6 μs. The Rabi oscillations contain two frequency components, which we attribute to a hyperfine interaction with a nuclear spin. The inset above shows the Rabi sequence of polarization, pulsed microwave (MW) excitation and optical readout. ( d ) Using the π /2 and π pulse durations from the Rabi measurement, we then applied a spin-echo sequence, determining the T 2 to be 230 μs. The inset above shows the Echo sequence of polarization, pulsed π /2 and π MW pulses, and optical readout. Full size image We use the relevant NV-nanocavity parameters to determine the possible impact of our system on established and potential future applications. NV-nanocavity system B lies in the strong Purcell regime with β =0.54, which would lead to a ~800-fold increase in entanglement generation rates between two distant NVs compared with present schemes without cavity enhancement, assuming the same collection efficiency as in previously reported experiments [20] ( Supplementary Note 4 ). For alternative collection schemes, it is possible to couple an optical fibre to a 1D cavity (similar to the one used in this work) through an intermediate waveguide with a total coupling efficiency of 85% (ref. 21 ), so even higher entanglement rates are achievable. Recently achieved quantum teleportation rates based on differentiating the excited spin states with high selectivity would also significantly benefit from this speed-up [22] . Another entanglement protocol relies on state-dependent reflectivity (resonant scattering) of an incoming photon on the cavity [23] . In this approach, the overall Purcell enhancement is important because it determines the probabilities of reflection and no reflection. If we neglect pure dephasing, we can set C , the cooperativity, equal to F and the reflection probability [23] is approximately given by 1−(1+4 F )/(1+4 F +4 F 2 ). Therefore, it is important to reach a high F >1. We show here a value of F ~1.2 in principle enabling the discussed entanglement scheme. However, we did not measure the dephasing properties and cannot confirm that we are operating in a regime without pure dephasing. These estimations indicate that coupling long-lived NVs to single-crystal diamond cavities is a critical step towards long-distance quantum entanglement and large-scale quantum networks. In conclusion, we have introduced a fabrication process for the creation of NV-nanocavity systems in the strong Purcell regime with consistently high Q factors, while preserving the long-spin coherence times of NVs [24] . These systems enable coherent spin control of cavity-coupled semiconductor qubits with coherence times exceeding 200 μs — an increase by 2 orders of magnitude over previously reported cavity-coupled solid-state qubits [8] , [18] , [19] . Such systems with specific NV-cavity coupling parameters can also be used for high-fidelity readout due to the modification of spin dynamics of cavity-coupled NVs [25] . Our on-chip architecture could be used to efficiently scale NV-nanocavity systems to many quantum memories connected via photons [26] , [27] , [28] , [29] . The membrane-transfer process introduced here is well-suited for building such networks as it allows the screening and subsequent integration of high-performance NV-nanocavity systems [30] , [31] , [32] , [33] into photonic integrated circuits equipped with MW circuits for multiple electron and nuclear spin control [34] , [35] , waveguide-integrated superconducting detectors [36] and low-latency logic devices for feed forward [37] . Spatial implantation of NVs into the mode field maximum or cavity fabrication around a single NV [38] appear promising to increase the NV-nanocavity overlap probability. Many of the schemes discussed above require coherent optical control of single or multiple NV spins in cavities that exhibit low spectral diffusion and lifetime-limited ZPL transitions; recent work on near-surface implanted NVs shows it is in principle possible to eliminate spectral diffusion even under 532 nm excitation [39] , [40] . With these advances, multiple NV-nanocavity systems operating in the strong Purcell regime and having long-spin coherence times would form scalable quantum memories for quantum repeaters [41] , spin-based microprocessors [42] and quantum networks [43] . Fabrication In the first fabrication step, high-purity ( 14 N<10 p.p.b.) single-crystal diamond plates were grown by MW-plasma-assisted CVD and were laser cut to a thickness of ~200 μm, where the area of the starting diamond sample falls in the range of 2 × 2 mm. The plates were polished down to ~5 μm membranes using a cast iron scaif. For the creation of NVs, a layer of nitrogen atoms was implanted at 80 keV energy and located ~100 nm from the surface. System A was implanted at a dosage of 5 × 10 10 15 N per cm 2 and system B at 5 × 10 11 15 N per cm 2 . The membrane was annealed in a MTI OTF-1500X-4 vacuum furnace (1.5 × 10 −6 mbar) for 2 h at 850 °C to mobilize lattice defects, which combine with 15 N atoms to form NV centres. Next, the membrane was turned over and thinned down to ~200 nm using plasma etching (Oxford ICP-RIE) with a mixture of chlorine and argon gases at a etch rate of ~2 μm h −1 . This recipe yielded a smooth surface (root-mean-square<1 nm) after 4.8 μm etching. The thinned membranes generally exhibited inhomogeneous thicknesses (100 to 300 nm) over hundreds of micrometers. The membrane was divided into tens of smaller pieces (each ~100 × 100 μm in size), which were transferred onto separate Si substrates using a polydimethylsiloxane (PDMS)-tipped tungsten probe. The Si PhC masks were designed and fabricated to match the thickness of each membrane, so that cavity resonances would fall near the NV’s ZPL, and then transferred onto the membranes using a PDMS-tipped probe. Oxygen plasma dry etching (Trion RIE at 20 sccm gas flow, 50 mTorr pressure and 100 W power) was used to transfer the pattern into the membranes. After the etch, little erosion was found on the Si PhC masks. A tungsten probe was used to remove Si masks from diamond membranes. Finally, an SF 6 isotropic dry etch removed the Si underneath to suspend the cavity structures. MW striplines were produced separately on intrinsic Si using a standard semiconductor fabrication process, followed by a lift-off step for metal deposition into the Si trenches. Finally, the diamond devices were integrated into the MW architecture using a PDMS-tipped probe. Low-temperature gas tuning Characterization of the optical properties of the sample at cryogenic temperatures was performed via PL measurements in a continuous flow He cryostat (CCS-XG-M/204N, Janis) at ~18 K. The sample was mounted inside the isolation vacuum and accessed through a window-corrected objective (LD Plan-Neofluar × 63, Zeiss numerical aperture=0.75). The NVs contained in the diamond cavity structures were excited with a 532-nm continuous-wave laser (Coherent Compass 315M). Fluorescence from the sample was collected in a confocal configuration and sent to fibre-coupled single photon detectors (SPCM-AQR, Perkin Elmer), while spectra were taken via free-space coupling into a spectrometer (Isoplane SCT320, Princeton Instruments). To spectrally tune the cavity mode into resonance with the ZPL, the cryostat was equipped with a nozzle near the cold finger for controlled gas flow onto the sample [44] . This feature can be used for condensation and ice formation of gas (for example, Xe) onto the sample, hence changing the effective refractive index of the diamond membrane. This refractive index change allows for spectrally red-tuning cavity resonances at a rate of ~8 pm s −1 . To take full advantage of this tuning technique, the cavities were designed to have resonances spectrally blue shifted from the ZPL. Xe gas can then be used to achieve precise in situ tuning of the cavity to overlap its resonance with the ZPL. We note that the cavity tuning was observed within seconds of the Xe being released, indicating no further gas dynamics. Reheating the sample to room temperature reverses the tuning. Using this procedure, we were able to repeatedly tune over a range of ~31 nm without significant degradation of the cavity Q . How to cite this article : Li, L. et al . Coherent spin control of a nanocavity-enhanced qubit in diamond. Nat. Commun. 6:6173 doi: 10.1038/ncomms7173 (2015).